South China Sea hydrological changes and Pacific Walker Circulation variations over the last millennium The relative importance of north–south migrations of the intertropical convergence zone (ITCZ) versus El Niño-Southern Oscillation and its associated Pacific Walker Circulation (PWC) variability for past hydrological change in the western tropical Pacific is unclear. Here we show that north–south ITCZ migration was not the only mechanism of tropical Pacific hydrologic variability during the last millennium, and that PWC variability profoundly influenced tropical Pacific hydrology. We present hydrological reconstructions from Cattle Pond, Dongdao Island of the South China Sea, where multi-decadal rainfall and downcore grain size variations are correlated to the Southern Oscillation Index during the instrumental era. Our downcore grain size reconstructions indicate that this site received less precipitation during relatively warm periods, AD 1000–1400 and AD 1850–2000, compared with the cool period ( AD 1400–1850). Including our new reconstructions in a synthesis of tropical Pacific records results in a spatial pattern of hydrologic variability that implicates the PWC. The tropical western Pacific is one of the major sources of heat and moisture for the globe and changes in hydrology of the region greatly impact global climate, even at high latitudes [1] . Tropical western Pacific rainfall varies in association with the seasonal march of the intertropical convergence zone (ITCZ)/monsoon coupled system. On interannual timescales, El Niño-Southern Oscillation (ENSO), and thus the strength and position of the PWC, also affects regional precipitation patterns [2] , [3] ( Supplementary Fig. S1 ). During El Niño events, the Walker circulation weakens and its rising limb shifts eastward away from the western Pacific warm pool. Consequently, the western Pacific receives less rainfall than under normal conditions ( Supplementary Fig. S1 ). The situation reverses during La Niña events [3] . Several studies suggest that hydrology of the tropical Pacific varies on centennial through millennial timescales. Compared with the recent warm period and the Medieval Climate Anomaly Period (MCA, ∼ AD 800–1300), the regions located at the northern limit of the ITCZ, including the East Asia continent [4] , [5] , were relatively dry during the time equivalent of the Little Ice Age (LIA, ∼ AD 1400–1850), whereas regions located closer to the southern limit of the ITCZ, including Indonesia, became wetter [6] , [7] , [8] . These variations suggest that the movement of the mean position of the ITCZ is a controlling influence for central and western Pacific hydrological changes on centennial timescale. However, recent work showing that these changes in the western Pacific were mirrored by hydrologic variability in the eastern tropical Pacific raises the possibility that changes in the PWC, whether due to ENSO or otherwise, may have also been an important influence on centennial-scale hydrological change in western Pacific during the past two millennia [8] . Additional data are required to test this hypothesis as to date there is no consensus on how the PWC or ENSO has evolved; for example, studies suggest both La Niña-like states/fewer El Niño events [9] , [10] , [11] and more El Niño events [12] , [13] during the MCA. To address the significance of changes in the PWC over the last millennium, we generated new records from Dongdao Island (16°39′–16°41′N, 112°43′–112°45′E), Xisha Islands, South China Sea ( Fig. 1 and Supplementary Fig. S2 ). The results suggest that this site consistently received less precipitation during relatively warm periods, AD 1000–1400 and AD 1850–2000, and more rainfall during the cool period ( AD 1400–1850). Including our new records in a synthesis of published records from the tropical Pacific rules out north–south ITCZ migration as the only mechanism of hydrologic variability at our core site. Our results suggest that changes in PWC profoundly influenced hydrology at our core site specifically, and in the tropics more generally, over the last millennium. 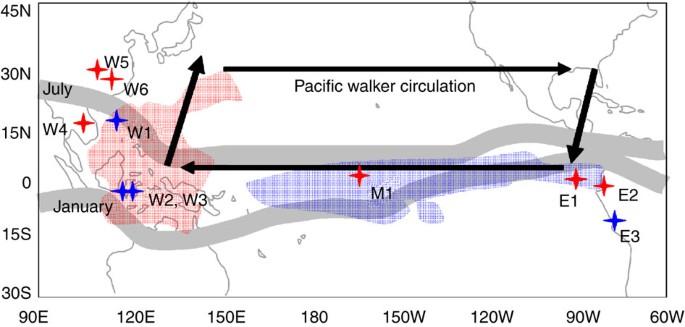Figure 1: Geographic context for the present study. Map showing modern locations of the ITCZ in July and January6. Locations of this study (W1, Dongdao Island) and other hydrology records near the northern limit of western Pacific ITCZ (W45, W54, W620). The dark cell represents the PWC. Areas in equatorial Pacific with correlation coefficient between SOI and precipitation above 0.6 are marked in red (named PA) and below −0.6 are marked in blue (named NA)3. Locations of the rainfall records in the PA of western Pacific (W1-our South China Sea records, W2-Indonesia6,7and W3-Indonesia8) and NA of eastern mid-tropical Pacific (M1-Washington Island17, E1-Galapagos13, E2-Ecuador12) are marked. Hydrology records from Peru (E310,11) are also indicated. Locations that were drier/wetter during the Little Ice Age (LIA,∼AD1400–1850) than during the MCA,∼AD800–1300) are marked in red/blue. Figure 1: Geographic context for the present study. Map showing modern locations of the ITCZ in July and January [6] . Locations of this study (W1, Dongdao Island) and other hydrology records near the northern limit of western Pacific ITCZ (W4 [5] , W5 [4] , W6 [20] ). The dark cell represents the PWC. Areas in equatorial Pacific with correlation coefficient between SOI and precipitation above 0.6 are marked in red (named PA) and below −0.6 are marked in blue (named NA) [3] . Locations of the rainfall records in the PA of western Pacific (W1-our South China Sea records, W2-Indonesia [6] , [7] and W3-Indonesia [8] ) and NA of eastern mid-tropical Pacific (M1-Washington Island [17] , E1-Galapagos [13] , E2-Ecuador [12] ) are marked. Hydrology records from Peru (E3 [10] , [11] ) are also indicated. Locations that were drier/wetter during the Little Ice Age (LIA, ∼ AD 1400–1850) than during the MCA, ∼ AD 800–1300) are marked in red/blue. Full size image Modern climatic characteristic in Dongdao Island The Dongdao Island is located in the northern margin of Indo-Pacific warm pool and near the northern limit of the ITCZ ( Fig. 1 and Supplementary Fig. S3 ) [6] , [14] . Thus seasonally, Dongdao Island receives most of its rainfall in boreal summer when the ITCZ moves to the Xisha area ( Supplementary Fig. S3 ). However, interannually, its precipitation is strongly related to the ENSO variability ( Supplementary Fig. S2 ). Instrumental records over the last 50 years from Xisha Islands show that rainfall is statistically correlated with the Southern Oscillation Index (SOI) [15] , [16] , with less precipitation during El Niño years ( Supplementary Fig. S1 and S4 ). This combination of seasonal and interannual variability is distinctly different from Indonesia, which is also dry during El Niño events, but wet during boreal winter, making it uniquely situated to test the role of the PWC on rainfall variability during the last millennium. The monthly mean latitude of ITCZ in South China Sea migrates between 3.3°N (February) and 17.9°N (August) ( Supplementary Fig. S3 ) [14] . Our study site (16.7°N) is located near the northern limit of the ITCZ; if ITCZ migration was the only factor influencing regional rainfall, one would expect Dongdao Island to be relatively dry during the LIA, when the ITCZ shifted southward (for example, Sachs [17] ). However, as we describe below, our records indicate wet conditions at that time. Lake sediment records and their hydrological implication We collected three lake sediment cores (DY2, DY4 and DY6) from the Cattle Pond on the Dongdao Island [18] ( Supplementary Figs S2 and S5 ). Detailed geochemical analyses showed that the three cores have similar lithologies (Lithology and chronology section in Methods and Supplementary Fig. S6 ). The present study is based mainly on the top 84, 58 and 112 cm ornithogenic sediment layers of DY2, DY4 and DY6 respectively, with a time span from AD 1024±30 to present (Lithology and chronology section in Methods and Supplementary Fig. S6 ). Here we present mean grain size results, along with previously reported carbon (δ 13 C) and oxygen isotopes (δ 18 O) of ostracode [18] (Sample collection and analysis section in Methods and Fig. 3). Variations in the grain size of lake sediments may be influenced by changes in lake level, paleoenvironmental zones of deposition, transport energy related to variations in wind, or rainfall [13] , [19] . As the water depth of the Cattle Pond remains steady due to the seepage between the pond and South China Sea ( Supplementary Information ), large-amplitude fluctuations of water levels cannot control mean grain size variations. Sediments in the Cattle Pond may be brought in by overland flows from sand barriers, which are composed of unconsolidated coral sand and covered by a few shrubs ( Supplementary Fig. S5 ). The precipitation on Dongdao Island is inherently associated with tropical storms, cyclones and even typhoons, and the sand layer around AD 1024 ( Supplementary Fig. S6 ) may indeed represent an overwash event. However, the lithological and geochemical characteristics [18] in the sediments deposited after AD 1024 are distinct from those in the sand layer and the observed mean grain size variations above that layer are unlikely linked with overwash events. The slopes of sand barriers are almost bare as the absence of organic remains in surface soils discourages plant growth. Thus, changes in the paleoenvironmental zones of deposition are probably insignificant in the Cattle Pond. Comparison to the instrumental record of the SOI indicates that mean grain size is most likely related to rainfall-controlled transport energy. The regression of the mean grain size from DY6 against 10-year averaged SOI values [15] , [16] yields a significant and positive correlation over the past 140 years ( r =0.58, P <0.01) ( Fig. 2 and Supplementary Fig. S7 ), with greater mean grain size corresponding to more precipitation on the island. Therefore, the change of transport energy associated with rainfall is probably the key factor controlling mean grain size variations. With increased rainfall, surface runoff increases; its greater erosion force brings larger terrestrial particles to the pond [19] . 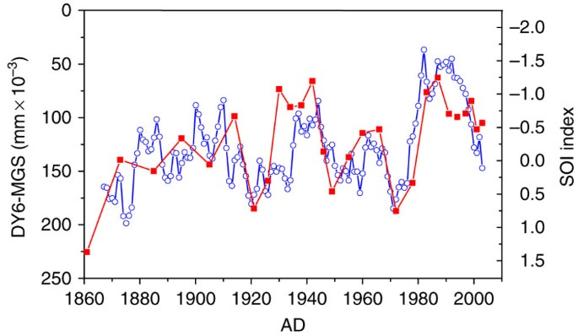Figure 2: Linking sediment grain size to SOI. Comparison of the DY6 sediment mean grain size (DY6-MGS) and 10-year-smoothing instrumental SOI15,16over the last 140 years. (SOI data come fromhttp://www.cgd.ucar.edu/cas/catalog/climind/SOI.signal.annstd.ascii). Figure 2: Linking sediment grain size to SOI. Comparison of the DY6 sediment mean grain size (DY6-MGS) and 10-year-smoothing instrumental SOI [15] , [16] over the last 140 years. (SOI data come from http://www.cgd.ucar.edu/cas/catalog/climind/SOI.signal.annstd.ascii ). Full size image Large fluctuations of mean grain size ( Fig. 3 ) suggest substantial hydrological changes on Dongdao Island over the last millennium. Very consistently, all three records (DY2, DY4 and DY6) show similar changes: relatively small grain size before ∼ AD 1400, increased grain size occurring during AD 1500–1700, and then reduced grain size over the last 150 years. Consistent with a runoff-transported mechanism, mean grain size gradually decreases from the water entrance to the deep centre of the pond (DY4>DY6>DY2, Supplementary Fig. S5 and Fig. 3 ). Based on the grain size records, we infer higher rainfall on the Dongdao Island approximately during the LIA ( ∼ AD 1400–1850), compared with the periods before and after. This inference is further supported by the records of δ 13 C and δ 18 O of ostracode shells in DY4 core [18] , which are also related to hydrological conditions ( Fig. 3 ). Both lower δ 18 O and δ 13 C values could be related to wetter conditions [18] . δ 18 O varied between −0.9‰ and −5.9‰ and δ 13 C ranged from −10.1‰ to −0.5‰ over the last millennium. Higher δ 18 O and δ 13 C values correspond to relatively small grain size, occurring during AD 1000–1400, whereas lower δ 18 O and δ 13 C values correspond to large grain size during AD 1500–1850. The δ 18 O and δ 13 C values for the last 150 years are probably unreliable as intact ostracode shells were not found in this section. Despite the common signal on centennial time scales, the mean grain size, δ 18 O, and δ 13 C proxy records do differ in some details. For instance, the mean grain size records show two distinct intervals of low values during the MCA, whereas δ 18 O does not ( Fig. 3 ). In addition to the low resolution of the δ 18 O record, the discrepancy may reflect different controlling factors for mean grain size and δ 18 O: grain size is mainly linked with precipitation, but δ 18 O values of ostracode shells can be affected by precipitation amount, lake evaporation and δ 18 O of precipitation [18] . Overall, although individual proxies might be complicated by additional factors, the main common signal on centennial time scales in the records of grain size, δ 18 O and δ 13 C of ostracode shells from the Dongdao Island reflects hydrological changes. 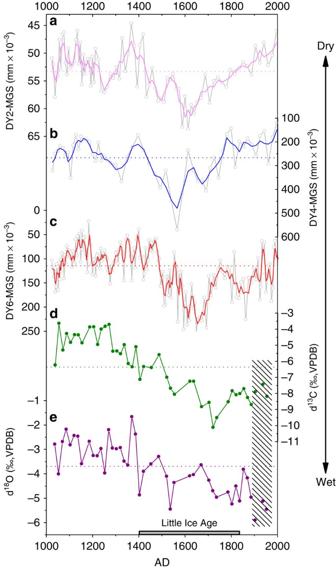Figure 3: Grain size and isotopic records of lake sediment cores from the Dongdao Island. Downcore mean grain size variations (3 points sliding average) of DY2 (a), DY4 (b) and DY6 (c); δ13C (d) and δ18O (e) of ostracode shells from DY4 core18. The isotope values were based on the Vienna PeeDee Belemnite (VPDB). Grey bars represent the approximate period of the LIA (∼AD1400–1850). The δ13C and δ18O data for the top 10 cm, indicated by diagonal shading, are questionable due to the absence of intact ostracode shells in this section. Figure 3: Grain size and isotopic records of lake sediment cores from the Dongdao Island. Downcore mean grain size variations (3 points sliding average) of DY2 ( a ), DY4 ( b ) and DY6 ( c ); δ 13 C ( d ) and δ 18 O ( e ) of ostracode shells from DY4 core [18] . The isotope values were based on the Vienna PeeDee Belemnite (VPDB). Grey bars represent the approximate period of the LIA ( ∼ AD 1400–1850). The δ 13 C and δ 18 O data for the top 10 cm, indicated by diagonal shading, are questionable due to the absence of intact ostracode shells in this section. Full size image Our records, together with hydrological reconstructions in the Makassar Strait of the western tropical Pacific [6] , [7] , [8] ( Supplementary Fig. S8 ) and from regions near the northern limit of ITCZ, including the East Asian continent and Vietnam [4] , [5] , [20] , indicate relatively wet conditions in the South China Sea and Indonesia and dry conditions on the East Asia continent approximately during the LIA ( Fig. 1 and Supplementary Fig. S8 ). Although the southward movement of the ITCZ during the LIA may explain the East Asian continent and Makassar Strait records [4] , [5] , [6] , [7] , [8] , the ITCZ mechanism is difficult to reconcile with wet LIA conditions inferred from our South China Sea records. A southward migration of the ITCZ should result in drier, not wetter, conditions in our South China Sea locality at ∼ 17°N near the northern limit of ITCZ [6] , [14] , [17] ( Supplementary Fig. S3 ). Furthermore, southward ITCZ migration cannot simultaneously explain the relatively dry LIA conditions in Vietnam [20] ( Fig. 1 ) and the relatively wet conditions in the South China Sea, as Vietnam and our study site are located at similar latitude and exhibit similar seasonal rainfall variability during the instrumental period. On the basis of the observation that our grain size records record the variability of ENSO/Walker circulation over the last 140 years ( Fig. 2 and Supplementary Fig. S7 ) and the difficulty of the ITCZ migration mechanism in explaining South China Sea hydrological changes of the last millennium, we propose that changes in PWC also profoundly influenced hydrology at our core site over the last millennium. This proposal implies that the wetter condition in the South China Sea during the most of the LIA reflects a strengthened and perhaps westward-shifted PWC compared with the MCA. To assess this hypothesis further, we compared our South China Sea records with hydrological records from other areas that are strongly influenced by ENSO/Walker circulation in modern climatology. The SOI is positively correlated with the precipitation over the Indo-Pacific warm pool and negatively correlated with the precipitation over the eastern and mid-tropical Pacific [3] . For convenience of discussion, we define the areas with correlation coefficient above 0.6 as PA or positive areas and below −0.6 as NA or negative areas [3] ; both PA and NA are deeply influenced by ENSO/walker circulation ( Fig. 1 ). 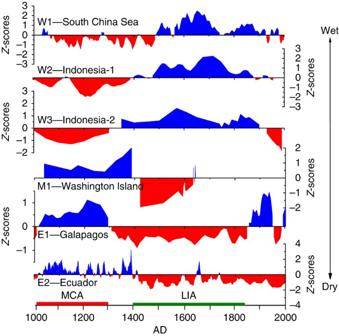Figure 4: Hydrological records from tropical Pacific. Hydrologic records from the PA of tropical western Pacific (W1—mean grain size of Cattle Pond sediments, W2—inferred seawater δ18O of Indonesia7and W3—δDwaxdata from Indonesia marine sediment for the C30n-acids8) and NA of eastern mid-tropical Pacific (M1—inferred lake salinity of Washington Island17, E1—sand percentages of El Junco lake sediment13and E2—red colour intensity of Laguna Pallcacocha sediment12). Site locations are given inFigure 1. All time series are three-points smoothed (except E2, 30-points smoothed) and normalized to standardZ-scores. StandardZ-scores are calculated according toZ=(X−V)/SD; hereXis original value,Vis the averaged value of the time series, and SD is the standard deviation of the time series. In all records, blue indicates relatively wet periods, and red relatively dry periods. As seen in Figure 4 , the records from PA [6] , [7] , [8] , [18] and NA [12] , [13] , [17] contained substantial multi-decadal variability characterized by an anti-phase oscillatory behaviour over the last millennium. During the LIA ( AD 1400–1850), proxy records indicate wetness in the western Pacific and aridity in the eastern-central tropical Pacific, suggesting an enhanced and westward PWC, with the opposite conditions prevailing during the MCA. We note, however, that according to the age models of the various records, hydrological changes were not synchronous throughout the tropical Pacific, and that in the South China Sea, the transition between dry and wet conditions might occur early in the LIA. Figure 4: Hydrological records from tropical Pacific. Hydrologic records from the PA of tropical western Pacific (W1—mean grain size of Cattle Pond sediments, W2—inferred seawater δ 18 O of Indonesia [7] and W3—δD wax data from Indonesia marine sediment for the C 30 n -acids [8] ) and NA of eastern mid-tropical Pacific (M1—inferred lake salinity of Washington Island [17] , E1—sand percentages of El Junco lake sediment [13] and E2—red colour intensity of Laguna Pallcacocha sediment [12] ). Site locations are given in Figure 1 . All time series are three-points smoothed (except E2, 30-points smoothed) and normalized to standard Z -scores. Standard Z -scores are calculated according to Z =( X − V )/SD; here X is original value, V is the averaged value of the time series, and SD is the standard deviation of the time series. In all records, blue indicates relatively wet periods, and red relatively dry periods. Full size image Many studies [9] , [10] , [11] , [12] , [13] have inferred tropical Pacific ENSO variability or mean state changes over the last millennium and beyond, but as discussed recently [8] the conclusions are controversial. Our results strongly suggest that changes in the PWC were an important influence on tropical hydrology. For the most part, a number of existing records, previously interpreted using the ITCZ migration hypothesis, can also be explained by a strong PWC during the relatively cold LIA period. These include records suggesting wetter Indo-Pacific region [6] , [7] , [8] , [18] ( Figs 1 and 4 ), drier central Pacific [17] ( Figs 1 and 4 ), and drier pan-Caribbean region [21] , [22] , [23] , [24] , [25] during the LIA. Sedimentary runoff indicators of hydrological change in lake sediments from the eastern equatorial Pacific, just south of the equator, suggest drier conditions during the LIA than MCA [12] , [13] , and are also consistent with a stronger westward-shifted PWC during the LIA [8] . We suggest that changes in the overall intensity or position of the PWC are likely to affect the frequency of storm deposits, whether or not they are directly associated with ENSO events. It should be noted, however, that in one of the same eastern Pacific lakes (El Junco, Lake Galápagos) hydrogen isotopes in lipids suggest wetter rather than drier conditions during the LIA [17] , and so there is still some uncertainty with respect to the hydrology of the eastern equatorial Pacific during the last millennium. On the other hand, a record of flood deposits near 13°S on the Peru Margin, indicating wet conditions during the LIA [10] , [11] , is also consistent with the PWC mechanism. This site experiences dry conditions during El Niño events ( Supplementary Fig. S1 ). Our new data strongly suggest that the PWC varied during the last millennia, and that these changes had a fundamental role in influencing tropical Pacific hydrology during the last millennium. As the ITCZ position and the PWC are to some extent coupled, ITCZ movements were also probably important. The challenge ahead is to reconcile evidence of a stronger, and perhaps westward-shifted PWC with that of more El Niño-like tropical Pacific sea surface temperature patterns during the LIA as compared with the MCA [26] , [27] . Whether, and if so how, inferred centennial-scale variations of the PWC during the last millennial are related to variations in interannual variability (ENSO) are also important questions for continued research [9] , [27] , [28] . Sample collection and analysis We collected three lake sediment cores named DY2 of 126 cm long, DY4 of 117 cm long and DY6 of 162 cm long from the Cattle Pond using PVC plastic gravity pipes of 12 cm diameter, during the field investigations in AD 2003 and 2008 ( Supplementary Figs S2 and S5 ). In the laboratory, the DY2, DY4 and DY6 cores were opened, photographed, described and then sectioned at 1 cm intervals for DY2 and DY4, and at 0.5 cm for DY6. Grain size was analysed for the top 83 cm of DY2, 58 cm of DY4, and 112 cm of DY6, above an interbedded coral sand layer (caused by a precipitous marine sedimentation event occurred at about AD 1024) [18] . All the subsamples were first sieved through a 2000-μm sieve and then approximately 0.5 g was taken for analysis at the Institute of Geology and Geophysics, Chinese Academy of Science, using a SALD-3001 laser particle analyser. The lithology and grain size results of DY2, DY4 and DY6 are presented in Supplementary Figure S6 . The δ 13 C and δ 18 O analyses were previously reported [18] . Dating methods Radiocarbon analyses for DY2 and DY4 cores were performed on terrestrial organic matter (plant caryopsis) and TOC ( Supplementary Table S1 ). A total of 16 samples were analysed using the Accelerator Mass Spectrometer facility at the Institute of Heavy Ion Physics in Beijing University ( Supplementary Table S1 ). The accelerator mass spectrometry radiocarbon dates are expressed in conventional 14 C yr BP . The determined radiocarbon dates were then calibrated into calendar years before present (cal. BP ) using the program OxCal version 4.4 and atmospheric data from Stuiver et al . (1998) [29] The dating results and age model of three cores are presented in Supplementary Table S1 and Figure S6 . The age model of the top 20 cm of DY6 was constructed by CRS (the constant rate of supply model) modelled 210 Pb ages ( Supplementary Table S2 ). 210 Pb (46.5 keV) and 214 Pb (295 and 352 keV) were measured in dried sediments from DY6 on a low-energy germanium detector (Institute of Polar Environment, University of Science and Technology of China, Hefei, Anhui, China). A 210 Pb chronology was constructed by assuming constant rate of supply and relating the exponential 210 Pb decay profiles with the cumulative dry mass–depth profiles as determined using bulk density measurements (DY6) and using a CRS model ( Supplementary Table S2 ). Lithology and chronology The 'Cattle Pond' on the Dongdao Island, Xisha Islands, South China Sea, is a crescent-shaped fresh lake, located within the southwestern sand barrier with a height of 6 m. It is about 150 m long and has a maximum width of 15 m ( Supplementary Figs S2 and S5 ). This pond is surrounded on three sides by elevated coral rocks that barricade the water flow. The lake water is completely fed by atmospheric precipitation and overland flow across a sand barrier ( Supplementary Fig. S5 ), and lost predominantly through evaporation and seepage. At present, the water depth remains steady at about 0.5 m probably due to the seepage between the Cattle Pond and South China Sea. Detailed geochemistry analysis in our previous study [18] showed that DY2 and DY4 sediment cores have similar lithologies. Three sediment units were identified on the basis of colour, LOI 950°C , CaO, LOI 550°C , TOC, TN and the presence of laminations [18] ( Supplementary Fig. S6 ). The bottom sediment units (Unit 3) of DY2 (126–96 cm) and DY4 (117–87 cm) consist of fragments of grey-white coral, shell and sandy gravels. These bottom sediments represent deposition in a lagoon environment, and they do not contain any plant remains. Above these sediments, both cores consist of ornithogenic sediments (Unit 1) with the exception of the well-sorted coral sand layers between 83 and 88 cm of DY2, and 58 and 69 cm of DY4 (Unit 2). The interbedded coral sand layer has a distinctly different lithology from the overlying and underlying sediments; it was formed around AD 1024 by a precipitous marine sedimentation event, an extraordinary washover deposition probably associated with an intense typhoon event, or even a tsunami ( Supplementary Fig. S6 ). Above the interbedded coral sand layer, the sediments displayed minor disturbance. The DY6 core has a lithology similar to DY2 and DY4 ( Supplementary Fig. S6 ), and the sediments above the interbedded coral sand layer are about 112 cm long, longer than that of DY2 (83 cm) and DY4 (58 cm). To eliminate the influence of the single precipitous marine sedimentation event, the present study is mainly based upon the top 84, 58 and 112 cm sediment layers of DY2, DY4 and DY6, respectively, with a time span from AD 1024 to present. (Detailed dating results and age model are given in Supplementary Fig. S6 and Table S1 .) How to cite this article: Yan, H. et al . South China Sea hydrological changes and Pacific Walker Circulation variations over the last millennium. Nat. Commun. 2:293 doi: 10.1038/ncomms1297 (2011).